Transcription factor IRF4 drives dendritic cells to promote Th2 differentiation Atopic asthma is an inflammatory pulmonary disease associated with Th2 adaptive immune responses triggered by innocuous antigens. While dendritic cells (DCs) are known to shape the adaptive immune response, the mechanisms by which DCs promote Th2 differentiation remain elusive. Herein we demonstrate that Th2-promoting stimuli induce DC expression of IRF4. Mice with conditional deletion of Irf4 in DCs show a dramatic defect in Th2-type lung inflammation, yet retain the ability to elicit pulmonary Th1 antiviral responses. Using loss- and gain-of-function analysis, we demonstrate that Th2 differentiation is dependent on IRF4 expression in DCs. Finally, IRF4 directly targets and activates the Il-10 and Il-33 genes in DCs. Reconstitution with exogenous IL-10 and IL-33 recovers the ability of Irf4 -deficient DCs to promote Th2 differentiation. These findings reveal a regulatory module in DCs by which IRF4 modulates IL-10 and IL-33 cytokine production to specifically promote Th2 differentiation and inflammation. Atopic asthma is an inflammatory pulmonary disease triggered by inhalation of innocuous antigens. While a variety of T-cell subsets are associated with specific asthmatic phenotypes, in atopic individuals, asthma is most commonly characterized by Th2-mediated responses. Th2 cells secrete IL-4, IL-5 and IL-13, which promote the hallmarks of allergy such as antibody class switching to IgE (immunoglobulin E), eosinophil recruitment, goblet cell mucus production and smooth muscle contraction [1] . Eliciting a Th2 response in the lungs is dependent on respiratory DCs; which are constitutively present in the lungs and airways and act as the primary antigen-presenting cell (APC) for lung allergic responses [2] , [3] . In addition to antigen presentation, cytokine production by DCs plays a critical role in promoting T-cell differentiation and shaping T-cell maturation. DCs producing IL-12 promote Th1 expansion in response to microbial stimuli [4] . While Il12 −/− DCs showed marked defect in generating Th1 responses, no change in Th2 responses were found. These data suggest that Th2 differentiation is not a default response in the absence of Th1-polarizing signalling from DCs, but rather that there are unique DC cytokines that promote Th2 differentiation [5] . Similarly, DCs are known to promote Th17 differentiation through secretion of the cytokines IL-23 and IL-1β [6] . Together, these data show that DCs mediate Th1 and Th17 differentiation through secretion of specific cytokines. However, DC cytokines that direct Th2 differentiation have yet to be elucidated [7] . Interestingly, IL-10 production by DCs has been linked with the promotion of Th2 differentiation [7] . Monocytes from allergic patients produced increased IL-10 and decreased IL-12 when stimulated with the house dust mite (HDM) antigen, Der p1, and promoted enhanced Th2 differentiation compared with those from non-allergic controls [8] . Our previous study, in mice, found that stimulation through FcγRIII (CD16) on LPS-activated DCs augmented IL-10 secretion while inhibiting IL-12. We determined that DC expression of FcγRIII and IL-10 was required for potent Th2 differentiation in vivo [9] . Similarly, utilization of Il10 −/− DCs showed loss of Th2 responses and dramatic Th1 skewing of naïve T cells in vitro , suggesting IL-10 from the priming APC might contribute to Th2 development [10] , [11] . These studies, using both animal models and asthmatic individuals, suggest that IL-10 production by DCs plays a critical role in the induction of Th2 differentiation during allergic responses and emphasize the importance of cytokine regulation in DCs in shaping the adaptive immune response. IL-33, a member of the IL-1β family, has recently emerged as an important player in the development of Th2 responses [12] . Two independent meta-analyses of GWAS data from asthmatic individuals identified highly associated SNPs in the IL-33 receptor locus ( IL1RL1;ST2) as well as the Il33 locus [12] . Il33 −/− mice and St2 −/− mice fail to develop strong Th2 responses following allergen sensitization and challenge. In addition to production by mast cells, macrophages and epithelial cells, IL-33 can be produced by DCs when activated [12] . We have found that IL-33 production from DCs augments the development of Th2 responses in an immune complex-induced model of lung inflammation [13] . Similarly, it has been suggested that IL-33 can promote an atypical Th2 response (IL-5/IL-13 only) when administered directly to naïve T cells in the presence of DCs without specific antigen [14] , [15] . While these findings emphasize the importance of IL-33 in the development of Th2-type responses, the mechanisms by which Il-33 is regulated and how it directly affects Th2 differentiation remain unclear. Interestingly, the transcription factor interferon regulatory factor 4 (IRF4) has been shown to bind to the Il-10 gene promoter and induce its expression in Th2 and Treg cells [16] , [17] , [18] , [19] . Unlike other members of the interferon regulatory factor (IRF) family, IRF4 is restricted to hematopoietic and adipocytic lineages, and activation of IRF4 expression is not induced by Type 1 or 2 interferon [20] , [21] , [22] . Rather, activation of IRF4 expression is regulated by NFκB and NFAT signalling modules downstream of the TCR in T cells, the BCR and CD40 in B cells, and by TLR4 in B and innate cells [23] , [24] , [25] , [26] . Accordingly, loss-of-function genetic experiments have shown that IRF4 plays an essential role in the differentiation of antigen-stimulated T and B cells, as well as the development of specific DC populations such as splenic CD11b + DCs [25] , [26] , [27] , [28] , [29] , [30] , [31] , [32] , [33] , [34] . Conditional deletion of Irf4 in CD11c + cells led to decreased development and survival of CD103 + CD11b + DCs in gut and CD11b + CD24 + DCs in lung. In both organs, lack of CD11b + DC subpopulations resulted in defective Th17 responses [33] , [34] . A recent study also shows a defect in skin CD301b + DC development in Irf4 conditional-deleted mice [35] . IRF4 has also been shown to function in DCs to modulate TLR signal transduction and regulate expression of CCR7 in skin-migratory DCs [36] , [37] , [38] . While these recent studies have emphasized an important role for IRF4 in DC development, there is currently limited research on how IRF4 may regulate the function and differentiation of mature DCs. Utilizing our previous findings on the role of FcγRIII signalling in the development of DCs that direct Th2 responses (referred to as DC Th2 ), we investigated transcriptional changes that occur upon DC Th2 differentiation. These studies reveal that IRF4 expression in DCs is augmented following FcγRIII signalling as well as after treatment with a Th2-promoting signal, HDM allergen. We developed DC-specific Irf4 conditional-deleted mice utilizing a different CD11c-cre system than previously reported [33] , [34] , [35] . Unlike other studies, the CD11c-cre positive Irf4 fl/fl mice in our studies have no defects in DC populations or proportions in the lungs, lymph node or spleen. Further, deletion of the Irf4 gene occurred after the pre-DC stage of development, thereby allowing for functional analysis of IRF4 in mature DC subsets. Conditional deletion of the Irf4 gene in CD11c + cells results in attenuation of allergic airway responses, but not pulmonary viral responses. Utilizing cell culture systems, we demonstrate that IRF4 functions in DCs to enable optimal Th2 differentiation, and that IRF4 targets and activates the cytokine genes encoding Il-10 and Il-33. Addition of exogenous IL-10 and IL-33 reconstitutes Irf4-deficient DC-driven Th2 differentiation. Together, these results suggest a pivotal role of IRF4-activated IL-10 and IL-33 production by DCs for the promotion of Th2 responses. Th2 stimuli augment IRF4 expression in DCs Previous research from our lab demonstrated that DCs deficient for FcγRIII ( Fcgr3 −/− ) failed to augment the development of Th2 responses, suggesting that FcγRIII signalling in DCs induces genes required for the priming of Th2 responses [9] , [13] . To elucidate candidate genes downstream of FcγRIII involved in the differentiation of DC Th2 , microarray analysis of B6 and Fcgr3 −/− BMDCs treated with OVA or OVA bound in immune complexes (OVA-IC) was performed. Interestingly, we identified Irf4 as a candidate transcription factor downstream of FcγRIII signalling in BMDCs, as it was upregulated in B6, but not Fcgr3 −/− DCs ( Fig. 1a ). This upregulation was validated by quantitative polymerase chain reaction ( Fig. 1b ). Expression of other IRF family member genes, Irf1, Irf2, Irf3 and Irf5 , were not affected by FcγRIII signalling, while Irf7 and Irf8 were downregulated in OVA-IC-treated DCs from both mouse strains ( Fig. 1a ). As we have previously reported, IL10 and IL33 were upregulated by OVA-IC treatment in B6 but not Fcgr3 −/− DCs, and IL12p35 was downregulated in DCs from both mouse strains [9] , [13] ( Fig. 1a ). Intracellular IRF4 staining demonstrated that IRF4 protein was augmented by OVA-IC stimulation of B6, but not Fcgr3 −/− BMDCs ( Fig. 1c ). We previously demonstrated that IC stimulation of the FcγRIII pathway for induction of DC Th2 could be mimicked with the combination of low-dose LPS and anti-FcγRIII/FcγRIIb (2.4G2) antibody [9] . This method was also sufficient to promote IRF4 expression in B6 BMDCs, but not in Irf4 −/− BMDCs ( Fig. 1d ). Thus, FcγRIII signalling, which induces DC Th2 development, resulted in upregulation of IRF4 expression in BMDCs. 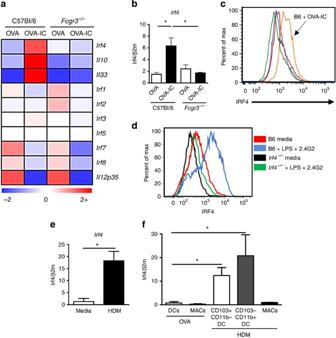Figure 1:Irf4expression is augmented in DCs by OVA-IC and HDM treatment. (a) BMDCs from C57Bl/6 orFcgr3−/−mice were grownin vitroand treated with either OVA or OVA-IC for 24 h. Three mice per group were used. RNA was isolated and run on an ABI mouse gene array. IRF family genes are shown (Irf6was below detection), as well as genes of interest:Il10,Il33,Il12p35. Data presented as relative expression fold-change. (b) Validation of microarray results by quantitative polymerase chain reaction ofIrf4expression in BMDCs following OVA or OVA-IC treatment. (c) BMDCs from B6 orFcgr3−/−mice were stimulatedin vitrowith OVA or OVA-IC for 24 h, then intracellular stained for IRF4 expression (orange, B6 OVA-IC; red, B6 OVA; green,Fcgr3−/−OVA; blue,Fcgr3−/−OVA-IC). (d) BMDCs from B6 orIrf4−/−mice were treated with LPS+2.4G2 or media control, and assayed for IRF4 intracellular expression. (e) BMDCs from B6 mice were stimulated with media or HDM for 16 h and assayed forIrf4expression. (f)B6mice were challenged i.t. with a single dose of either OVA or HDM. Three hours later pulmonary DCs (including some monocyte CD11c+, SSClo) and macrophage (CD11c+, SSChi) populations were sorted and assayed for expression ofIrf4. HDM-treated samples were further separated into CD103+DC or CD11b+DC/monocyte populations. Data represent the mean ±s.e.m. and tested for significance by (a) Analysis of variance (b–f) Student’st-test; *P<0.05. Data are representative of three independent experiments, with three or more replicates in each experiment. Figure 1: Irf4 expression is augmented in DCs by OVA-IC and HDM treatment. ( a ) BMDCs from C57Bl/6 or Fcgr3 −/− mice were grown in vitro and treated with either OVA or OVA-IC for 24 h. Three mice per group were used. RNA was isolated and run on an ABI mouse gene array. IRF family genes are shown ( Irf6 was below detection), as well as genes of interest: Il10 , Il33 , Il12p35 . Data presented as relative expression fold-change. ( b ) Validation of microarray results by quantitative polymerase chain reaction of Irf4 expression in BMDCs following OVA or OVA-IC treatment. ( c ) BMDCs from B6 or Fcgr3 −/− mice were stimulated in vitro with OVA or OVA-IC for 24 h, then intracellular stained for IRF4 expression (orange, B6 OVA-IC; red, B6 OVA; green, Fcgr3 −/− OVA; blue, Fcgr3 −/− OVA-IC). ( d ) BMDCs from B6 or Irf4 −/− mice were treated with LPS+2.4G2 or media control, and assayed for IRF4 intracellular expression. ( e ) BMDCs from B6 mice were stimulated with media or HDM for 16 h and assayed for Irf4 expression. ( f ) B6 mice were challenged i.t. with a single dose of either OVA or HDM. Three hours later pulmonary DCs (including some monocyte CD11c + , SSC lo ) and macrophage (CD11c + , SSC hi ) populations were sorted and assayed for expression of Irf4 . HDM-treated samples were further separated into CD103 + DC or CD11b + DC/monocyte populations. Data represent the mean ±s.e.m. and tested for significance by ( a ) Analysis of variance ( b – f ) Student’s t -test; * P <0.05. Data are representative of three independent experiments, with three or more replicates in each experiment. Full size image HDM allergen, one of the most common triggers for asthma and allergies, has previously been found to promote DC Th2 differentiation [39] . To determine whether IRF4 was also induced following stimulation with HDM, BMDCs were treated with HDM overnight. qPCR demonstrated that HDM effectively augmented Irf4 expression in BMDCs ( Fig. 1e ). To test whether pulmonary DCs and monocytes responded similarly to HDM challenge in vivo , B6 mice were intratracheally (i.t.) treated with a single dose of HDM or a control protein, OVA, and lung DC/monocyte and macrophage subsets were sorted using flow cytometry for RNA analyses. Irf4 was augmented in the CD103 + DCs (CD11c + MHCII + Auto lo CD103 + CD11b − ) and the CD11b + DC/monocyte population (CD11c + MHCII + Auto lo CD103 − CD11b + ) from HDM-challenged mice compared with OVA-challenged mice, but not in the macrophage population (CD11c + Auto hi ) ( Fig. 1f ). Together, these data demonstrate that Th2-inducing stimuli promote Irf4 upregulation in DCs in vitro as well as in vivo . IRF4 in CD11c cells is necessary for Th2 lung inflammation Irf4 conditional-deleted mice were generated using a CD11c-cre promoter ( Irf4 fl/fl CD11cCre ) to analyse the functional importance of IRF4 in respiratory DCs in Th2 inflammatory responses. Germline Irf4 −/− mice and conditional deletion of Irf4 in CD11c + cells are known to lead to defects in DC subpopulation development [30] , [33] , [34] , [35] . Since our Irf4 fl/fl CD11cCre mice were bred with a different CD11c-Cre strain than those previously reported [33] , [34] , [35] , [40] , [41] , we first determined whether there were defects in DC development in our Irf4 fl/fl CD11cCre strain. We compared DC subpopulations in the Irf4 fl/fl CD11cCre, Irf4 fl/fl and Irf4 −/− mice, and found that as previously reported, Irf4 −/− mice have a defect in the lymph node CD11c + MHCII + migratory DCs ( Fig. 2a ), as well as a defect in the splenic CD8 − negative DC subset ( Fig. 2b ) [30] , [31] , [36] . Interestingly, the Irf4 fl/fl CD11cCre mice had no major defects in either of these DC populations in the lymph node or spleen ( Fig. 2a,b ). Further using generally accepted markers [3] , [42] , [43] , [44] , we found no significant differences in the lungs of Irf4 fl/fl and Irf4 fl/fl CD11cCre mice in macrophages (CD11c + Siglec-F + ), eosinophils (CD11c − Siglec-F + ), CD103 + DCs (CD11c + MHCII HI Siglec-F − CD103 + CD11b − ), monocyte-derived DCs (moDCs; CD11c + MHCII HI Siglec-F − CD103 − CD11b + CD64 + Fc ∈ RI int ) or CD11b + DCs (cDCs; CD11c + MHCII HI Siglec-F − CD103 − CD11b + CD64 − Fc ∈ RI − ) ( Fig. 2c ). Similarly, Irf4 fl/fl and Irf4 fl/fl CD11cCre mice showed no differences in lung T cell or granulocyte proportions ( Supplementary Fig. S1 ). 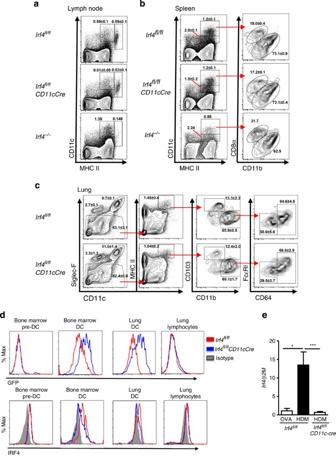Figure 2:Irf4fl/flCD11cCremice have normal DC populations. NaïveIrf4fl/flandIrf4fl/flCD11cCremice were killed and assayed for dendritic cell populations in the inguinal lymph node (a), spleen (b) and lung (c). AnIrf4−/−mouse is included in LN and spleen to show known defects in DC populations. (d) Intracellular IRF4 staining or GFP expression from bone marrow pre-DCs (Lin−CD11clo/+CD11b−MHCIIlo/−Flt3+) and DCs (CD11c+MHCII+) and lung lymphocytes and DCs (CD11c+MHCII+Autolo) from naïveIrf4fl/flandIrf4fl/flCD11cCre. (e) HDM-challenged lung DC and monocytes (CD11c+ Autolo) fromIrf4fl/florIrf4fl/flCD11cCremice assayed for IRF4 message. Statistics represent mean ±s.e.m. and include at least three mice for each group and tested for significance by Student’st-test; *P<0.05; ***P<0.001. Figure 2: Irf4 fl/fl CD11cCre mice have normal DC populations. Naïve Irf4 fl/fl and Irf4 fl/fl CD11cCre mice were killed and assayed for dendritic cell populations in the inguinal lymph node ( a ), spleen ( b ) and lung ( c ). An Irf4 −/− mouse is included in LN and spleen to show known defects in DC populations. ( d ) Intracellular IRF4 staining or GFP expression from bone marrow pre-DCs (Lin − CD11c lo/+ CD11b − MHCII lo/− Flt3 + ) and DCs (CD11c + MHCII + ) and lung lymphocytes and DCs (CD11c + MHCII + Auto lo ) from naïve Irf4 fl/fl and Irf4 fl/fl CD11cCre . ( e ) HDM-challenged lung DC and monocytes (CD11c+ Auto lo ) from Irf4 fl/fl or Irf4 fl/fl CD11cCre mice assayed for IRF4 message. Statistics represent mean ±s.e.m. and include at least three mice for each group and tested for significance by Student’s t -test; * P <0.05; *** P <0.001. Full size image To confirm deletion of IRF4 in mature DCs, we first utilized analysis of GFP expression, which can be turned on by expression of CD11c-cre-EGFP or by excision of the first two exons of IRF4 caused by Cre expression. We find that mature DCs from the bone marrow and from the lung uniformly expressed high levels of GFP, while bone marrow pre-DCs (Lin − CD11c lo/+ MHCII lo/− CD11b − Flt3 + ) and lung lymphocytes were largely negative for GFP expression. To further validate our model, intracellular IRF4 staining was used to confirm loss of IRF4 protein in Irf4 fl/fl CD11cCre DCs compared with Irf4 fl/fl DCs in the lung and bone marrow while showing no change in IRF4 expression in lung lymphocytes or bone marrow pre-DCs ( Fig. 2d ). Additionally, respiratory DC/monocytes from Irf4 fl/fl CD11cCre mice failed to upregulate Irf4 expression after HDM challenge thereby demonstrating that Irf4 expression was effectively deleted in the CD11c + respiratory DCs and monocytes in these mice ( Fig. 2e ). These data suggest that while IRF4 is important for the development of particular DC subsets, the CD11c-promoter segment used in our CD11c-cre transgenic mice induces deletion of Irf4 after DC progenitors have passed the stage at which IRF4 function is required in their development. To determine the function of IRF4 in CD11c + cells in the development of Th2 inflammatory responses in vivo, Irf4 fl/fl CD11cCre or Irf4 fl/fl mice were sensitized and challenged with HDM i.t. on days 0, 7, 8, 9 and 10, then assayed for development of airway inflammation. Interestingly, while Irf4 fl/fl mice exhibited a strong Th2 inflammatory response, Irf4 fl/fl CD11cCre mice failed to recruit eosinophils, CD4 T cells or CD8 T cells to the bronchoalveolar lavage fluid (BAL) and lungs ( Fig. 3a,b ). Histological sections from the lungs showed decreased cellular infiltration and mucus production in Irf4 fl/fl CD11cCre mice compared with the Irf4 fl/fl controls ( Fig. 3c ). Importantly, Irf4 fl/fl CD11cCre mice showed a dramatic defect in the percentage of IL-5 + CD4 T cells and a decreased total number of IL-5 + and IL-13 + CD4 T cells in the lungs of sensitized and challenged mice ( Supplementary Fig. S2 ). HDM-specific cytokine secretion by lung T cells also confirmed a decreased Th2-cytokine production profile ( Fig. 3d ). This defect was Th2 specific, as there was no change in the number or HDM-specific response of T cells producing the Th1 cytokine, IFNγ ( Fig. 3d,e ). Importantly, neither were these results due to changes in migratory DC populations, as similar number of resident and migratory DCs were found in the mediastinal lymph nodes following HDM challenge ( Supplementary Fig. S3A ). Interestingly, IgE responses in HDM sensitized and challenged mice showed no significant difference between Irf4 fl/fl and Irf4 fl/fl CD11cCre mice ( Supplementary Fig. S3B ). Finally, in a second HDM challenge model in which systemic sensitization was first given by i.p. injection of HDM and Alum prior to HDM i.t. challenge, Irf4 fl/fl CD11cCre mice also demonstrated a reduced Th2 inflammatory response ( Supplementary Fig. S4 ). Together these data demonstrated that in the absence of IRF4 in CD11c + cells, Th2 responses and the resulting lung inflammation is severely attenuated. 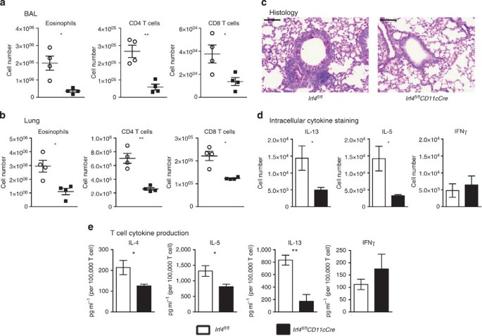Figure 3: IRF4 in DCs is necessary for development of Th2-mediated HDM allergic airway inflammation. Irf4fl/fl(open circles) andIrf4fl/flCD11cCre(black squares) mice were sensitized and challenged with HDM by i.t. instillation. Mice were killed 3 days after the final challenge and assayed for inflammation and development of Th2 responses. Cell infiltration of eosinophil, CD4 and CD8 T cells in the (a) BAL and (b) lung digests were calculated using flow cytometry. (c) Lung histology was sectioned and stained with PAS to show cell infiltration and mucus production in the airway. (d) CD4 T cells from the lungs were restimulated with PMA/ionomycin and assayed by intracellular IL-5, IL-13 and IFNγ cytokine staining. (e) T cells from the lungs of sensitized and challenged mice were restimulated with HDM in the presence of irradiated APCs for antigen-specific cytokine production. Histology bar, 100 μM. Data represent the mean ±s.e.m. and tested for significance by Student’st-test; *P<0.05; **P<0.01. Data are representative of three independent experiments each. Figure 3: IRF4 in DCs is necessary for development of Th2-mediated HDM allergic airway inflammation. Irf4 fl/fl (open circles) and Irf4 fl/fl CD11cCre (black squares) mice were sensitized and challenged with HDM by i.t. instillation. Mice were killed 3 days after the final challenge and assayed for inflammation and development of Th2 responses. Cell infiltration of eosinophil, CD4 and CD8 T cells in the ( a ) BAL and ( b ) lung digests were calculated using flow cytometry. ( c ) Lung histology was sectioned and stained with PAS to show cell infiltration and mucus production in the airway. ( d ) CD4 T cells from the lungs were restimulated with PMA/ionomycin and assayed by intracellular IL-5, IL-13 and IFNγ cytokine staining. ( e ) T cells from the lungs of sensitized and challenged mice were restimulated with HDM in the presence of irradiated APCs for antigen-specific cytokine production. Histology bar, 100 μM. Data represent the mean ±s.e.m. and tested for significance by Student’s t -test; * P <0.05; ** P <0.01. Data are representative of three independent experiments each. Full size image To determine whether the defect in Th2-mediated responses in Irf4 fl/fl CD11cCre mice was specific for Th2 responses or broadly applicable to other CD4 T-cell responses in the lung, mice were infected with influenza (H1N1, PR8). This infection results in both a strong CD8 T cell and a Th1-biased CD4 T-cell response. Both the pulmonary CD103 + and CD103 − CD11b + DCs/monocytes have been shown to contribute to the activation of CD4 and CD8 T cells during an influenza infection [45] , [46] . Following infection, Irf4 fl/fl and Irf4 fl/fl CD11cCre mice showed similar susceptibility to the influenza infection ( Fig. 4a ). Accordingly, at the peak inflammatory response on day 8, no difference was observed in weight loss ( Fig. 4b ), in CD4 and CD8 T cell numbers in the lungs ( Fig. 4c ), in the cytokine responses of these T cells ( Fig. 4d ), or in lung histologic inflammation ( Fig. 4e ). Thus, IRF4 appears dispensable in CD11c + cells for the priming of Th1 responses to viral infection. These data suggest that IRF4 has a specific regulatory function that is required in DCs for the induction of Th2-specific responses to allergens. 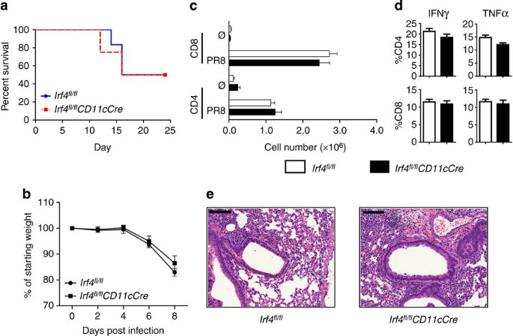Figure 4:Irf4-deficient DCs mount potent pulmonary T-cell responses to influenza infection. (a)Irf4fl/flandIrf4fl/flCD11cCremice were infected with influenza (PR8) and survival was measured for 25 days. (b) Weight was measured following infection until killing on day 8. (c) CD4 and CD8 T cell numbers in the lungs of infected mice on day 8 following infection. (d) Percentage of IFNγ and TNFα-positive CD4 and CD8 T cells in the lungs of infected mice at day 8. (e) H&E stain of lung histology from mice 8 days post infection,Irf4fl/fl(left)Irf4fl/flCD11cCre(right). Histology bar, 100 μM. Data represent the mean±s.e.m. and tested for significance by Student’st-test. Data are representative of three independent experiments each. Figure 4: Irf4 -deficient DCs mount potent pulmonary T-cell responses to influenza infection. ( a ) Irf4 fl/fl and Irf4 fl/fl CD11cCre mice were infected with influenza (PR8) and survival was measured for 25 days. ( b ) Weight was measured following infection until killing on day 8. ( c ) CD4 and CD8 T cell numbers in the lungs of infected mice on day 8 following infection. ( d ) Percentage of IFNγ and TNFα-positive CD4 and CD8 T cells in the lungs of infected mice at day 8. ( e ) H&E stain of lung histology from mice 8 days post infection, Irf4 fl/fl (left) Irf4 fl/fl CD11cCre (right). Histology bar, 100 μM. Data represent the mean±s.e.m. and tested for significance by Student’s t -test. Data are representative of three independent experiments each. Full size image Modulation of IRF4 in DCs regulates Th2 differentiation To address whether the attenuated Th2 response to HDM allergen challenge in Irf4 fl/fl CD11cCre mice was due to defects in Th2 skewing, BMDCs from Irf4 fl/fl and Irf4 fl/fl CD11cCre mice were activated by HDM ( Fig. 5a ) or LPS ( Fig. 5b ), and utilized to present OVA peptide to OTII TCR-Tg T cells in vitro . T cells activated by Irf4 fl/fl CD11cCre BMDCs showed significant decreases in Th2 responses upon restimulation, independent of the adjuvant used to activate DCs. In contrast, there were little or no detectable changes in the Th1 (IFNγ) or Th17 (IL-17) cytokine responses, implicating a role for IRF4 in BMDCs in the promotion of Th2 responses in vitro . This was not due to differences in MHCII and CD86 expression in the Irf4 fl/fl and Irf4 fl/fl CD11cCre BMDCs following LPS stimulation or in their induction of OTII T-cell proliferation ( Supplementary Fig. S5 ). It has recently been argued that Flt3L-derived DCs mimic the conventional CD11b + DC population more closely than GM-CSF-derived cultures; therefore, we also tested the role of IRF4 in CD11b + Flt3L-derived BMDCs in promoting Th2 responses. We found that OTII T cells stimulated with Flt3L-BMDCs from Irf4 fl/fl CD11cCre mice had decreased Th2 differentiation compared to OTII T cells stimulated with Irf4 fl/fl Flt3L-BMDCs ( Fig. 5c ). Interestingly, Irf4 fl/fl CD11cCre Flt3L-BMDCs resulted in a significant augmentation of IFNγ and IL-17 secretion by OTII T cells. Irf4 fl/fl CD11cCre BMDCs and Flt3L-DCs treated overnight with HDM showed no dramatic defects in the surface expression of molecules involved in DC:T-cell interactions (CD80, CD86, PIR-B, OX40L, PD-L1, PD-L2, CCR7, ST2 and CD40), suggesting IRF4 regulates Th2 differentiation through alternative pathways ( Supplementary Fig. S6A,B ). We next tested whether sustained expression of high levels of IRF4, in combination with DC activation, could promote the differentiation of DC Th2 cells. To perform this experiment, we compared BMDCs derived from control mice or mice harbouring a tet-inducible allele of Irf4 ( Irf4 -inducible mice on the Irf4 +/+ background) treated with doxycycline, a high affinity analogue of tetracycline [29] , [47] . Activated BMDCs from Irf4- inducible mice increased IRF4 expression when treated with doxycycline ( Fig. 5d ). Remarkably, Irf4 -inducible BMDCs demonstrated that sustained expression of high levels of IRF4 in BMDC enhanced Th2-cytokine production (IL-5 and IL-13), while decreasing Th1 cytokine (IFNγ) production ( Fig. 5e ). Overall, these findings emphasize the importance of IRF4 in promoting the differentiation of DC Th2 cells, and suggest that an inflammatory milieu or signals that preferentially augment IRF4 expression in DCs could skew the ensuing T-cell response. 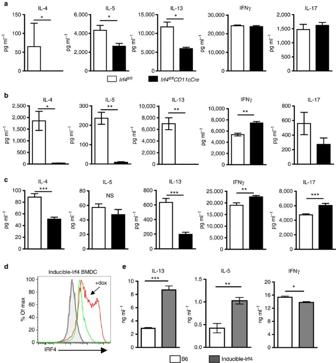Figure 5: IRF4 in DCs controls the differentiation of Th2 cellsin vitro. GM-CSF-induced BMDCs activated with either (a) 25 μg ml−1HDM or (b) 10 ng ml−1LPS and (c) sorted CD11b+Flt3L-induced DCs activated with 25 μg ml−1HDM were used to activate OTII T cells in the presence of 1 ug ml−1OVAp. T cells were collected after 5 days and restimulated with anti-CD3 antibody for cytokine analysis. (d) BMDCs from inducibleIrf4mice were grownin vitroand activated with or without addition of doxycycline and assayed for IRF4 expression 24 h later. (e) BMDCs from C57BL/6 or inducibleIrf4mice were generated and used to stimulate OTII T cells in the presence of doxycycline and assayed for cytokine secretion as described above. Data represent the mean ±s.e.m. and tested for significance by Student’st-test; *P<0.05; **P<0.01; ***P<0.001; NS, not significant. Data are representative of two independent experiments each, with 3–8 replicates per experiment. Figure 5: IRF4 in DCs controls the differentiation of Th2 cells in vitro . GM-CSF-induced BMDCs activated with either ( a ) 25 μg ml −1 HDM or ( b ) 10 ng ml −1 LPS and ( c ) sorted CD11b + Flt3L-induced DCs activated with 25 μg ml −1 HDM were used to activate OTII T cells in the presence of 1 ug ml −1 OVAp. T cells were collected after 5 days and restimulated with anti-CD3 antibody for cytokine analysis. ( d ) BMDCs from inducible Irf4 mice were grown in vitro and activated with or without addition of doxycycline and assayed for IRF4 expression 24 h later. ( e ) BMDCs from C57BL/6 or inducible Irf4 mice were generated and used to stimulate OTII T cells in the presence of doxycycline and assayed for cytokine secretion as described above. Data represent the mean ±s.e.m. and tested for significance by Student’s t -test; * P <0.05; ** P <0.01; *** P <0.001; NS, not significant. Data are representative of two independent experiments each, with 3–8 replicates per experiment. Full size image IRF4 directly activates Il10 and Il33 gene expression in DCs Our studies have found that DC Th2 induction by FcγRIII signalling leads to the production of IL-10 and IL-33 by DCs ( Fig. 1a ) [9] , [13] . Expression of these cytokines was also elevated by treatment with HDM in BMDCs from control mice ( Fig. 6a ). Strikingly, HDM treatment of BMDCs ( Fig. 6a ) and CD11b + MHCII + Flt3L-DCs ( Fig. 6b ) from Irf4 fl/fl CD11cCre mice failed to induce expression of Il10 and Il33 transcripts. 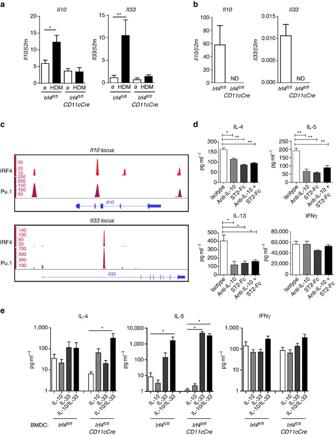Figure 6: IRF4 promotes Th2 differentiation through upregulation of IL-10 and IL-33 in DCs. (a)Irf4fl/flandIrf4fl/flCD11cCreBMDCs were stimulated with media alone or HDM overnight and assayed forIl-10andIl-33gene expression. (b) CD11b+Flt3L-DCs fromIrf4fl/flandIrf4fl/flCD11cCremice were treated with HDM overnight and assayed forIl-10andIl-33expression. (c) BMDCs from WT mice were stimulated with LPS and assayed by ChIP-seq for binding sites of IRF4 and Pu.1.Il-10andIl-33genes are shown. (d) HDM-activated WT BMDCs were used to stimulate OTII T cells in the presence of 1 μg ml−1OVAp and addition of isotype control, anti-IL-10, ST2-Fc or both. OTII cells were collected 5 days later and restimulated for cytokine secretion. (e)Irf4fl/flandIrf4fl/flCD11cCreBMDCs were used to differentiate OTII T cells in the presence of HDM, OVAp and addition of media or recombinant IL-10, IL-33 or IL-10+IL-33. T cells were collected and restimulated for cytokine production. Data represent the mean ±s.e.m. and tested for significance by Student’st-test; *P<0.05; **P<0.01. Data are representative of two or three independent experiments with 3–6 replicates per experimental group. Figure 6: IRF4 promotes Th2 differentiation through upregulation of IL-10 and IL-33 in DCs. ( a ) Irf4 fl/fl and Irf4 fl/fl CD11cCre BMDCs were stimulated with media alone or HDM overnight and assayed for Il-10 and Il-33 gene expression. ( b ) CD11b + Flt3L-DCs from Irf4 fl/fl and Irf4 fl/fl CD11cCre mice were treated with HDM overnight and assayed for Il-10 and Il-33 expression. ( c ) BMDCs from WT mice were stimulated with LPS and assayed by ChIP-seq for binding sites of IRF4 and Pu.1. Il-10 and Il-33 genes are shown. ( d ) HDM-activated WT BMDCs were used to stimulate OTII T cells in the presence of 1 μg ml −1 OVAp and addition of isotype control, anti-IL-10, ST2-Fc or both. OTII cells were collected 5 days later and restimulated for cytokine secretion. ( e ) Irf4 fl/fl and Irf4 fl/fl CD11cCre BMDCs were used to differentiate OTII T cells in the presence of HDM, OVAp and addition of media or recombinant IL-10, IL-33 or IL-10+IL-33. T cells were collected and restimulated for cytokine production. Data represent the mean ±s.e.m. and tested for significance by Student’s t -test; * P <0.05; ** P <0.01. Data are representative of two or three independent experiments with 3–6 replicates per experimental group. Full size image In CD4 T cells, IRF4 has been shown to bind to the Il10 promoter and to activate expression of the Il10 gene [16] , [17] , [19] . Whether IRF4 targets and regulates Il10 and Il33 in DCs are unknown. To determine whether IRF4 targets these cytokine genes in BMDCs, we examined ChIP-seq data sets for IRF4 and its binding partners PU.1 and BATF ( Fig. 6c ) [48] . Binding of these transcription factors was analysed in LPS stimulated BMDCs and normalized to input. At the Il10 locus, we found that IRF4 and PU.1 co-bound several regions including at the proximal promoter and within the second intron. At the Il33 locus, we detected co-binding of IRF4 and PU.1 within the first intron. BATF did not show enriched binding on these gene loci in BMDCs. Each of the IRF4 and PU.1 co-bound regions were unbound in input samples and each contained canonical Ets-IRF composite elements (GEO GSE44388). Together, these data demonstrate that IRF4 targets and activates the transcription of the Il10 and Il33 genes. IL-10 and IL-33 recovers Th2 skewing by IRF4-deficient DCs The significance of IL-10 and IL-33 expression in promoting Th2 differentiation in coculture assay was tested using ST2 (IL-33R) Fc fusion protein and IL-10 neutralizing antibody in WT BMDC-OTII coculture assays. Interestingly, blockade of either IL-10 or IL-33 was sufficient to inhibit Th2 differentiation in our coculture assay ( Fig. 6d ). Since IRF4-deficient DCs were found to have defects in both Il10 and Il33 expression, we tested whether the absence of these cytokines controlled defects in Th2 skewing by IRF4-deficient DCs. Accordingly, Irf4 fl/fl and Irf4 fl/fl CD11cCre BMDCs were used to present OVA peptide to OTII T cells in vitro in the presence of exogenous IL-10 and IL-33. Interestingly, addition of IL-33 alone was sufficient to recover IL-5 production by T cells stimulated with Irf4 fl/fl CD11cCre DCs ( Fig. 6e ). However, addition of both IL-10 and IL-33 together was required to rescue IL-4 production by the OTII cells stimulated with Irf4 fl/fl CD11cCre BMDCs. No effect of the two cytokines was found on OTII T cell production of IFNγ ( Fig. 6e ). Importantly, the effects of IL-33 in coculture experiments were not due to contamination by ILC2 cells since using our methodology for T-cell enrichment, ILC2s are undetectable (<0.002%) [13] . Together, these data suggest that IRF4-induced IL-10 and IL-33 production by DCs promotes the differentiation of Th2 cells. The aim of this study was to discover transcriptional regulators in DCs that promote DC Th2 differentiation, which in turn promote the development of Th2-mediated allergic responses. Using an unbiased microarray approach, Irf4 was identified as a candidate gene that could participate in the programming of DC Th2 cells. Activating DCs with the Th2-inducing stimuli, immune complexes or HDM, upregulated IRF4 expression. Importantly, IRF4 was shown to be necessary for DC-mediated Th2-type responses in the lung, but dispensable for Th1 responses to influenza infection. IRF4 bound and activated Il10 and Il33 genes in DCs, and addition of these cytokines was able to restore defects in the IRF4-deficient DCs in promoting Th2 differentiation in vitro . Thus, we have provided new and compelling evidence demonstrating the role of IRF4 in DC Th2 differentiation and allergic Th2 responses in mice through promotion of Th2-promoting cytokine production. IRF4 has been shown to be a key transcription factor in the development and function of various immune cells, including B cells, T cells and macrophages [21] , [49] , [50] . Disruption of the Irf4 gene in mice revealed a role for IRF4 in the development of specific subsets of CD11b + DCs in the spleen, lymph nodes, lung, small intestine and skin [30] , [31] , [33] , [34] , [35] , [36] . These studies lead to the hypothesis that IRF4 was necessary for the development or maintenance of CD11b + DC populations and further studies showing that CD11b + DCs are necessary for the promotion of a variety of CD4-mediated responses [33] , [34] , [35] . Interestingly, spleen, lymph node and lung defects were not observed in our Irf4 fl/fl CD11cCre animals ( Fig. 2 ). These mice were produced by breeding the Irf4 fl/fl mice with the CD11c-Cre-Gfp mice developed by Chervonsky and colleagues that contains 5 kb of the 5′ Cd11c -promoter region [25] , [40] . Since Irf4 −/− mice deplete subsets of DCs while the Irf4 fl/fl CD11cCre do not, the CD11c-Cre promoter employed in our mouse model is not sufficiently activated to cause deletion of IRF4 until after the pre-DC stage of development ( Fig. 2 ). Therefore, unlike previous studies on the role of CD11b + DC-deficient mice [33] , [34] , [35] in which the pertinent DC population was missing or greatly reduced, our conditional-deleted mice had no defect in DC populations or numbers, thereby uniquely allowing for analysis of the specific role of IRF4 in mature DCs in vivo . Several studies have demonstrated that in murine models of allergic lung disease CD11b + conventional DCs are the primary mediator of the allergic responses [3] , [51] , [52] . This DC subset expresses IRF4 in both humans and mice [53] , [54] . Treatment of human DCs with the Th2-promoting stimulus TSLP also augments IRF4 through a STAT5-dependent pathway [55] , [56] . Both GM-CSF and IL-4 treatment can promote upregulation of IRF4 in mouse CD11b + DCs, mouse bone marrow macrophages and human monocyte-derived DCs [53] , [54] , [57] , [58] . In fact, in human monocyte-derived DCs, IRF4 is both self-amplifying and directly regulated by STAT and NFκB signalling pathways [54] . While these studies provide a correlation between signals that promote DC Th2 and those that promote IRF4 activation, our findings now establish that IRF4 activation in DCs is a key regulator of DC Th2 differentiation. We show that IRF4 in CD11c + cells is functionally necessary for the development of Th2-mediated inflammatory responses in the lung ( Fig. 3 ). Interestingly, we did not find defective IgE production following HDM challenge in Irf4 fl/fl CD11cCre mice. This is an important observation, because it suggests that while the Th2 response is defective in the lungs (reduced Th2 cells and eosinophilia), the follicular T helper cell (Tfh) response, which is responsible for promoting IgE class switching in B cells during Th2-type responses, is intact and capable of promoting IgE antibody responses [59] , [60] . Interpretation of these findings along with previous data show that while IRF4 is necessary for DC differentiation, activated DCs utilize IRF4 specifically in the promotion of Th2 responses, and not for the development of Th1 ( Fig. 4 ) or Tfh responses ( Supplementary Fig. S3B ). Through gain and loss–of-function studies, we find that IRF4 activation correlates with differentiation of DCs into DC Th2 ( Fig. 5 ). Irf4 -deficient DCs (GM-CSF and Flt3L-derived) induced Th2 differentiation less efficiently than wild-type DCs in vitro , while DCs expressing elevated IRF4 levels promoted Th2 differentiation more efficiently than wild-type DCs. It is interesting that even though GM-CSF- and Flt3L-derived DCs have been argued to be important mediators of unique populations of in vivo DCs, we find that both in vitro -derived GM-CSF BMDCs and Flt3L-DCs are dependent on IRF4 to promote Th2 differentiation [44] , [61] , [62] . In the presence of sustained IRF4 expression, functional DC Th2 differentiation was enhanced and even occurred at the expense of eliciting a Th1 phenotype. In contrast to previous publications showing that IRF4-dependent DCs regulated Th17 responses, our data suggest that IRF4 does not directly regulate the promotion of Th17 differentiation [33] , [34] . Our study did not examine Th17-specific responses in vivo , therefore it is possible that using a direct Th17 promoting antigen such as Aspergillus fumigatus may yield a different result. Whether the expression dynamics of IRF4 in DC cells functions to dictate alternate cell fates (DC Th2 vs DC Th1/Th17 ) during cellular activation, as has been shown for B cells (GC B cells vs plasma cells), will be an important area of future study. Collectively, we propose that depending on the nature and amount of the allergic stimulants, responding DC cells that transiently express IRF4 would generate minor IL-10 and IL-33 secretion, and blunted Th2 differentiation resulting in mild exacerbation. In contrast, responding DCs that sustainably express high levels of IRF4 would lead to durable IL-10 and IL-33 secretion, vigorous Th2 differentiation and would result in more severe Th2 lung inflammation. IL-33 is known to be an important cytokine for the promotion of Th2 responses. While airway epithelium is a major source of IL-33, we and others observed that IL-33 production by DCs and alveolar macrophages can contribute to the development of airway disease [12] , [13] . Molecular analyses of HDM-activated GM-CSF- and Flt3L-BMDCs demonstrated that expression of Il10 and Il33 genes are directly promoted by IRF4 ( Fig. 5a–c ). Importantly, complementation of Irf4 fl/fl CD11cCre BMDCs with recombinant IL-33 and IL-10 to cultures fully recovered the impaired Th2 development caused by loss of IRF4. IRF4 plays a multifaceted role in the function of DCs, and therefore it is possible that other IRF4-dependent mechanisms independent of cytokine promotion may influence the development of Th immune responses. Similarly, the other regulators of DC Th2 differentiation may be involved in the induction of Th2 responses. Nevertheless, our findings show a novel and exciting pathway by which IRF4 promotes Th2 responses through IL-10 and IL-33. The findings of IL-10 promoting Th2 differentiation support previous reports showing a role for IL-10 from stimulating APCs for the promotion of Th2 responses [9] , [63] , [64] , [65] . Independent of currently known pathways of IL-33 production from epithelial cells and its actions on innate lymphoid cells and mast cells in the lungs, our findings underscore the importance of IL-33 production from DCs in directly promoting Th2 cells and Th2-mediated inflammation. DCs are at the interface between the innate and adaptive immune response, and represent a primary target for development of therapeutics in a variety of disease models, including asthma. Collectively, our data have revealed a key role for IRF4 in DCs in the promotion of allergic disease, and highlight a separate role for IRF4 distinct from its function in DC development. Rapid induction of IRF4 following allergic stimulation promoted the production of IL-10 and IL-33 in order to drive Th2-specific responses. These findings identify IRF4 as a key regulator of DC Th2 development and suggest its potential as a valuable therapeutic target for the treatment of allergic disorders and disease. Mice Fcgr3 −/− (B6.129P2-Fcgr3 thm1Sjv /J), OTII (B6.Cg-Tg(TcraTcrb)425Cbn/J) and conditional Irf4 mutant ( Irf4 fl/fl ; B6.129S1-Irf4 tm1Rdf /J) mice were purchased from The Jackson Laboratory (Bar Harbor, Maine, USA). Irf4 fl/fl mice were bred to CD11c-cre-GFP mice (C57Bl/6 J-Tg(Itgax-cre,-EGFP)4097Ach/J), which were developed and kindly provided by Dr Alexander Chervonsky [40] (University of Chicago). In these mice, GFP is a marker of both the CD11c-Cre expression as well as effective deletion of IRF4 (ref. 25 ). While the CD11c + cells were uniformly GFP positive, GFP expression in non-CD11c + cells was negligible. Irf4 -inducible and Irf4 −/− mice have been previously described [47] . B6 (C57Bl/6) mice were purchased from Harlan Industries (Indianapolis, IN). For in vivo experiments, mice were co-housed, blinded by ear tagging, mixed gender and used at age 6–12 weeks for all experiments. All mice were bred and housed in specific pathogen-free facilities maintained by the University of Chicago Animal Resource Center. The studies described conform to the principles set forth by the Animal Welfare Act and the National Institutes of Health guidelines for the care and use of laboratory animals in biomedical research and were approved by the University of Chicago Institutional Animal Care and Use Committee. Bone marrow-derived DC cultures BMDCs were cultured as previously described [9] . This protocol utilizes total bone marrow cells and cultures with GM-CSF-supplemented media on bacteriological-coated plates to allow for suspension of DCs. Harvested cells were analysed by flow cytometry for purity of CD11c + CD11b + ≥85%. Flt3L-derived DC cultures were grown as previously described [66] , briefly, bone marrow was isolated and grown in vitro for 7–10 days in complete RPMI-media supplemented with 200 ng ml −1 hFlt3L (PeproTech). BMDCs (5 × 10 5 ) were cultured on 24- or 96-well plates with stimulation (25 μg ml −1 HDM, 50 μg ml −1 OVA, 50 μg ml −1 OVA-IC, 200 ng ml −1 doxycycline (Sigma), 1 ug ml −1 OVAp, or 10 ng ml −1 LPS (Invitrogen)) as described in Results. IL-10 and IL-33 inhibition assays used 10 μg ml −1 anti-IL-10 antibody (JES5-16E3, Biolegend) and 1 μg ml −1 ST2-Fc (R&D Systems). OVA-IC was prepared by mixing 4:1 ratio of anti-OVA rabbit serum (Sigma) to OVA at 37 °C for 30 min as previously described [13] . Control samples were made by passing sera over protein G column to deplete IgG present and then mixing the aliquot with OVA as control samples. DC activation was measured by flow cytometry following 8 h of culture in media with 10 ng ml −1 LPS or overnight treatment with 25 μg ml −1 HDM. Microarray and ChIP-Seq RNA isolated from treated C57Bl/6 and FcγRIII −/− BMDCs were run on an ABI Mouse Genome Survey Microarray (Applied Biosystems) by the University of Chicago Functional Genomics Facility. All microarray gene expression data in this study are available from the Gene Expression Omnibus (GEO), accession number GSE44388 . ChIP was performed and analysed as previously described [48] . Input controls found no detectable binding on the l10 and Il33 loci (data not shown). This data series is available from GEO accession number GSE40727 , and the SubSeries is part of SuperSeries GSE40483. HDM-induced allergy model House dust mite (Greer Laboratories) in phosphate-buffered saline (PBS) was administered to mice i.t. on day 0 with 100 μg of HDM and again on day 7, 8, 9 and 10 with 25 μg HDM, then killed on day 13. For systemic HDM protocol, mice were sensitized intraperitoneally on day 0 with 40 μg HDM in 4 mg Alum (Sigma), then challenged i.t. on day 7 with 100 μg HDM and killed on day 11. At killing, BAL was performed by delivering 0.8 ml cold PBS into the airway via a tracheal cannula and gently aspirating the fluid. The lavage was repeated four times. Lungs were dissociated by mechanical mincing followed by digestion with 150 U ml −1 Collagenase I (Invitrogen) in 10 ml for 30 min. Samples were then washed and red blood cells were lysed. Spleens and lymph nodes were collected and cells liberated by mechanical dissociation. Cells were counted using a hemacytometer and the percentage of CCR3 + eosinophils, CD4 + T cells and CD8 + T cells in the BAL were determined using flow cytometry. Lung peribronchial inflammation was scored blindly on a scale of 0–4. T-cell cytokine production Lung samples from inflamed mice were isolated as described. Samples were then incubated in the presence of irradiated T cell-depleted splenocytes in the presence of 25 μg ml −1 HDM for 48 h. Supernatants were frozen and assayed for cytokine production by Millipore multiplex cytokine kit following manufacturer’s instructions. Influenza model PR8 (influenza A, H1N1) was kindly provided by Amanda L. Marzo, Rush University. Ten thousand p.f.u. of influenza was instilled intranasally and mice were monitored daily for weight loss. Mice were assessed for inflammation 8 days following infection. Flow cytometric analysis In brief, 5 × 10 5 cells were suspended in 50 μl of fluorescence-activated cell sorting buffer (PBS containing 0.1% sodium azide and 1% BSA) and labelled with specific antibodies. Antibodies used include: anti-CCR7 (4 μg ml −1 , 4B12), CD3 (1 μg ml −1 , 145-2C11), CD4 (125 ng ml −1 , GK1.5), CD8 (250 ng ml −1 , 53-6.7), CD86 (500 ng ml −1 , GL-1), IL-13 (2 μg ml −1 , eBio13A), IFNγ (1 μg ml −1 , XMG1.2), PD-L1 (2 μg ml −1 , J43), PD-L2 (2 μg ml −1 , TY25), TNF-α (2 μg ml −1 , MP6-XT22) (eBiosciences), CD40 (2 μg ml −1 , 3/23), CD80 (500 ng ml −1 , 16-10A1), Siglec-F (500 ng ml −1 , E50-2440) (BD Biosciences), IL-5 (2 μg ml −1 , TRFK5), CD11c (1 μg ml −1 , N418), CD11b (250 ng ml −1 , M1/70), I-A/I-E (1 μg ml −1 , M5/114.15.2), CD103 (500 ng ml −1 , 2E7), CD64 (2 μg ml −1 , X54-5/7.1), Fc ∈ RIα (2 μg ml −1 , Mar1), OX40L (2 μg ml −1 , RM134L), ST2 (4 μg ml −1 , DIH9) (Biolegend), CCR3 (1 μg ml −1 , 83101), PIR-B (2 μg ml −1 , 326414) (R&D Systems) and unconjugated goat anti-IRF4 (4 μg ml −1 , Santa Cruz) with secondary Donkey anti-goat IgG-PE (500 ng ml −1 , Abcam) were used. For intracellular staining, cells were fixed with 1% paraformaldehyde and permeabilized with 0.5% saponin in PBS containing 0.1% BSA. After fixation and permeabilization, cells were incubated with specified antibodies. Flow cytometric analysis was performed on a LSRFortessa or LSRII (BD Biosciences), and the data were analysed with FlowJo software (Tree Star). Cell sorting experiments were performed using FACSAriaII (BD Biosciences). All instruments are maintained by the University of Chicago Flow Cytometry and Antibody Technology Core Facility. T-Cell enrichment and in vitro stimulation assays Lymph nodes were collected from OTII mice and passed through nylon wool columns to deplete B cells and DCs. Nonadherent cells were collected and assayed for T-cell purity of greater than 90%. For proliferation studies, OTII cells were stained with CFSE (Invitrogen) following manufacturer’s instructions and incubated with activated DCs in the presence of 1 μg ml −1 OVAp. For in vitro differentiation assays, DCs and T cells were cocultured at a 1:10 ratio in 96-well round bottom plates with described adjuvants and OVAp. T cells were collected 5 days later and restimulated on anti-CD3 (2C11)-coated plates for cytokine production. Histology Lungs were removed from mice after BAL and fixed in 4% formalin for 48 h. Samples were then sectioned sagittally, embedded in paraffin and cut in 5-μm sections. Sections were stained with hematoxylin and eosin for analysis of cellular infiltrate or with periodic acid Schiff for analysis of mucus production. Quantitative real-time polymerase chain reaction RNA from cells or tissue was isolated using an RNeasy Micro or Mini Kit (Qiagen). cDNA was synthesized using Superscript III Reverse Transcriptase Kit (Invitrogen) following the manufacturer’s instructions. cDNA samples were assayed using Power Sybr Green PCR master mix (Applied Biosystems) and run using an ABI 7300 thermalcycler (Bio-Rad). qRT–PCR cycling conditions were optimized for each primer set but in general, included an initial denaturation at 95 °C for 2′, followed by 40 cycles of 94 °C for 30′′, 56 °C for 30′′, and 72 °C for 3′. Relative abundance of gene targets was determined by comparative CT (cycle threshold) number normalized against tested B2M comparative CT. Primers used were: IRF4, forward 5′-AGATTCCAGGTGACTCTGTG-3′, reverse 5′-CTGCCCTGTCAGAGTATTTC-3; IL-10, forward 5′-GCCAAGCCTTATCGGAAATGATCC-3′, reverse 5′-CACAGGGGAGAAATCGATGACAG- 3′; IL-33, forward 5′-CTGCGTCTGTTGACACATT-3′, reverse 5′-CACCTGGTCTTGCTCTTGGT-3′; β2 M, forward 5′-CATACGCCTGCAGAGTTAAGCA-3′,reverse 5′-GATCACATGTCCGATCCCAGTAG-3′. Statistical analysis Statistics were calculated using GraphPad Prism software. All data are represented as the mean ±s.e.m. where P -values<0.05 were considered significant (* P <0.05; ** P <0.01; *** P <0.001; NS, not significant). Student’s t -tests were used to analyse data sets with only two groups. Analysis of variance tests with post hoc Tukey tests were used to determine significance when more than two groups were being compared. How to cite this article : Williams, J. W. et al. Transcription factor IRF4 drives dendritic cells to promote Th2 differentiation. Nat. Commun. 4:2990 doi: 10.1038/ncomms3990 (2013).